Green chemistry and nanofabrication in a levitated Leidenfrost drop Green nanotechnology focuses on the development of new and sustainable methods of creating nanoparticles, their localized assembly and integration into useful systems and devices in a cost-effective, simple and eco-friendly manner. Here we present our experimental findings on the use of the Leidenfrost drop as an overheated and charged green chemical reactor. Employing a droplet of aqueous solution on hot substrates, this method is capable of fabricating nanoparticles, creating nanoscale coatings on complex objects and designing porous metal in suspension and foam form, all in a levitated Leidenfrost drop. As examples of the potential applications of the Leidenfrost drop, fabrication of nanoporous black gold as a plasmonic wideband superabsorber, and synthesis of superhydrophilic and thermal resistive metal–polymer hybrid foams are demonstrated. We believe that the presented nanofabrication method may be a promising strategy towards the sustainable production of functional nanomaterials. Sprinkling a drop of water onto a hot skillet is an everyday event that was first investigated by Leidenfrost [1] . When a water drop touches a hot plate whose temperature is much higher than the boiling point of water, the part of the drop which comes in contact with the hot surface vapourizes immediately and the drop levitates on its own vapour. Using water, Leidenfrost [1] found remnant solid was left on the heated surface. In our previous work, we found that this remnant solid has the form of nanoparticulate wires and rings left by a small drop loaded with a precursor, mobilized by the Leidenfrost effect [2] , [3] . Starting with the Leidenfrost temperature itself, which has been described by a large number of terms, including minimum film boiling, rewetting temperature, quenching temperature and others, a wide variety of investigations have been performed to explore the Leidenfrost phenomenon. The physical picture emerging from these investigations suggests that fast vapourization and expansion of the superheated part of the layer adjacent to the hot substrate provide the driving force for the observed phenomenon [4] , [5] , [6] , [7] , [8] . It is worth noting that the Leidenfrost temperature is not a unique property of the liquid and might be changed by the properties of the surface, for example, surface roughness and wettability [9] , [10] . In our previous work [3] we postulated the existence of an overheated state in the Leidenfrost droplet, which has been utilized as a chemical reactor. For example, water droplets containing dissolved zinc acetate or silver nitrate yielded zinc oxide and metallic silver nanoclusters respectively. These observations raised many questions about the phenomenon and the origins of the nanoparticles formation. For instance, we could not prove where and how the particles were formed, nor could we explore the role of water in the synthesis. Here we show our progress with the Leidenfrost phenomenon; trying to answer those questions, establishing the first steps towards the understanding of the 257-year-old phenomenon, demonstrating a green chemistry lab inside the levitated droplet and simultaneously implementing it in the design of functional materials. For instance, we report experimental proof of the electrostatic nature of the Leidenfrost droplet and its implementation as an overheated and charged chemical reactor inside a levitated droplet. The fabrication of nanomaterials, creation of nanoscale coatings and design of plasmonic porous metal and hybrid foam could all be realized in a levitated Leidenfrost drop. Thermal gradient and overheated zone in the Leidenfrost drop With sufficiently brief contact between the cold droplet and the hot surface, impulse heating of the contact layer occurs, which leads to superheating of this layer. Following a brief incubation period, fast evaporation and expansion of the vapourized molecules near the surface forces the outer water layers to move away, resulting in the levitation of the droplet, as shown in Fig. 1a–c . This method was used to determine the Leidenfrost temperature on various substrates in our experiments, including aluminum, silicon oxide and commercial silicon. 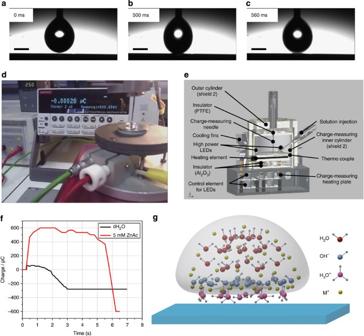Figure 1: Levitation and charge separation at Leidenfrost temperature. Steps of producing the vapour cushion (Leidenfrost effect) with a drop of water held by a needle and placed on a hot aluminum plate illustrate the approaching of the droplet to the preheated surface (a) and show a time frame of the incubation state (b), and the levitation state (c). (a–c) Scale bar, 1 mm. (d) Foreground: water drop levitating on the hot surface with the needle immersed in it, background: charge measurement output panel showing negative charge measured in the drop. (e) Lab-built set-up of the closed apparatus used for accurate measurements of the charge generation under Leidenfrost condition. Charge can be measured at the top, the bottom and on the walls of the inner cylinder. The device is controlled by the software ‘National Instruments LabView’. (f) Charge curves of deionized water and 5 mM zinc acetate solution measured inside the droplet show at the initial contact no charge, followed by an increase of positive charge and finally a slow continuous increase of negative charge, whereas zinc acetate enhanced the charge separation. (g) 3D sketch of the postulated mechanism for green nanochemistry with a Leidenfrost drop: fast evaporation generates an overheated zone, which along with the self-ionization of water at the liquid-vapour interface gives rise to a local increase in metal (M+) and hydroxyl (OH−) ion concentrations. The increase in hydroxyl ion concentration is attributed to loss of the hydronium ions (H3O+) to the vapours; hence the basic condition is satisfied. Figure 1: Levitation and charge separation at Leidenfrost temperature. Steps of producing the vapour cushion (Leidenfrost effect) with a drop of water held by a needle and placed on a hot aluminum plate illustrate the approaching of the droplet to the preheated surface ( a ) and show a time frame of the incubation state ( b ), and the levitation state ( c ). ( a – c ) Scale bar, 1 mm. ( d ) Foreground: water drop levitating on the hot surface with the needle immersed in it, background: charge measurement output panel showing negative charge measured in the drop. ( e ) Lab-built set-up of the closed apparatus used for accurate measurements of the charge generation under Leidenfrost condition. Charge can be measured at the top, the bottom and on the walls of the inner cylinder. The device is controlled by the software ‘National Instruments LabView’. ( f ) Charge curves of deionized water and 5 mM zinc acetate solution measured inside the droplet show at the initial contact no charge, followed by an increase of positive charge and finally a slow continuous increase of negative charge, whereas zinc acetate enhanced the charge separation. ( g ) 3D sketch of the postulated mechanism for green nanochemistry with a Leidenfrost drop: fast evaporation generates an overheated zone, which along with the self-ionization of water at the liquid-vapour interface gives rise to a local increase in metal (M + ) and hydroxyl (OH − ) ion concentrations. The increase in hydroxyl ion concentration is attributed to loss of the hydronium ions (H 3 O + ) to the vapours; hence the basic condition is satisfied. Full size image In all of our experiments, the Leidenfrost state was observed at a temperature above 230 °C, which is approximately the same as the temperature required for homogenous phase transitions of water at 1 atm [11] . At temperatures lower than that, the stable state in the Leidenfrost phenomenon was not observed. Although the vapour layer underneath the droplet is heated by various mechanisms [12] , including induced convection to a mean temperature approximately equal to the heated substrate, the temperature of the droplet is generally assumed to be approximately at the boiling point of water, that is, 100 °C (ref. 10 ). As the thermal conductivity of water is sufficiently low, and owing to the expected evaporative cooling of the levitated droplet, a temperature gradient in the droplet should be established with an overheated region at the liquid–vapour interface, a task that has not been proved so far. Although an exact temperature determination at a multiphase interface is always a difficult task [13] , we determined a temperature gradient in a single droplet by using an infrared thermography camera (see Supplementary Fig. S1 ) as a non-contact temperature measurement tool, capable of detecting radiation in the far-infrared range. Indeed, a vertical and horizontal temperature gradient is found inside the drop and the drop maintains a global evaporation as predicted [14] , and now ascertained by our measurement. Although the skin of the drop is much colder than the interior, the interface of the levitated drop bears an overheated zone as we postulated, which points to the existence of the two-phase regions (liquid/vapour). It should be borne in mind that there is no sharp partition at the interface between the superheated vapour/hot liquid underneath the Leidenfrost droplet, rather both regions are joined by what we called ‘overheated zone’, whose boundaries and temperature, which could even exceed 100 °C, are still unknown and have to be determined. Indeed, a recent report on the Leidenfrost phenomenon [15] shows that the vapour layer under a Leidenfrost drop is not uniform, which further supports our finding. There is a significant temperature difference between the base (warm) and the top surface (cool) of the levitated drop, indicating a possible thermoelectric effect and, hence, a charge separation event [16] . Charge chemistry and green chemistry in a Leidenfrost drop Water, which undergoes a fast phase expansion, shows different characteristics, including enhanced self-ionization and charge separation, which has been shown by Volta and George [17] , and further studied by Faraday [18] and Lenard [19] . Further investigations [20] , [21] , [22] , [23] revealed the generation of a positively charged steam under the conditions of rapid evaporation. Although the level of understanding for the charge separation phenomenon is insufficient for its quantitative description [24] , our interest, here, is to show whether this effect appears with the Leidenfrost drop. For that purpose, a metal tungsten tip was connected to a grounded electrometer and the aluminum metal surface was preheated to 250 °C. The aluminum surface was isolated from the grounded hot plate with an insulator ceramic. The tip was placed at a distance of 300 μm from the hot surface. As shown in Fig. 1d ( Supplementary Movie 1 ), the Leidenfrost drop was negatively charged during the levitation. It is worth mentioning that no charges were registered with a deionized water drop at room temperature or even at boiling temperature. Two sets of experiments on an insulated preheated ceramic were carried out to eliminate any effect from the substrate and to differentiate between the charges inside the drop and vapour. The tip was set above the drop to register only the charge of the vapour phase, which resulted in only positive charges; their magnitude increased each time when a new droplet was added ( Supplementary Movie 2 ). However, on placing the tip at a distance of 1 mm from the preheated, insulated ceramic and applying small droplets of deionized water (that is, the tip enters the levitated droplet at the upper part), only negative charges were registered ( Supplementary Movie 3 ). To optimize the accuracy of the measurement, that is, to prevent the access to air or impurities, also to avoid charge leakage, the measurement of the levitated droplet was repeated in a closed lab-built apparatus controlled by the National Instruments LabView software ( Fig. 1e ). For the charge measurement, the tip was placed at distance of 300 μm from the hot surface and a drop was injected to the hot aluminum surface, that is, T =250 °C. When a drop of deionized water falls on the preheated surface, it undergoes a fast evaporation followed by levitation as explained previously and showed in Fig. 1a–c . In this process, charges separate during the fast evaporation. As shown in Fig. 1f , transitory positive charges were registered at the beginning, followed by permanent increasing of negative charges during the levitation until the charge curves reached a negative saturated value. Indeed, no charges were registered during the initial period, which correspond to the first contact between the cold droplet and the hot surface, indicating that the fast evaporation and steam generation caused by the fast rupture of the layer adjacent to the hot substrate are essential for the charge separation process as demonstrated by Lenard [19] , and Gilbert and Shaw [24] . Furthermore, the charge generation under the Leidenfrost condition was enhanced by an order of magnitude when a salt solution droplet was used (see Fig. 1f ). It already confirmed that ions at high salt concentrations can destroy the natural hydrogen-bonded network of water and thus enhance the self-ionization similar to increased temperature or pressure [25] . This effect is governed at the overheated interface by the fast phase expansion. Here the water density and the solubility of ions are considerably reduced, thus giving rise to a local increase of the ion concentration. Hence, self-ionization and, subsequently, the charge separation of the water are enhanced. Our proof-of-concept experiments indicated that overheating, thermal gradients and charge separation are generic under Leidenfrost conditions. Although we explored the electrostatic nature of the levitated droplet, our findings are also important to enhance our comprehension of not yet fully understood phenomena of the Leidenfrost dynamics, such as deformation, vibration, internal circulation, oscillation and rotation inside the Leidenfrost drop. However, here we restrict ourselves to explore the phenomena solely for nanochemistry. For instance, the difference in measured charges in the droplet and vapour under the Leidenfrost condition manifest the earlier finding [17] , [18] , [19] , [20] , [21] , [22] of the charge separation and shows its occurrence with the Leidenfrost droplet. Accordingly, we postulate that the fast evaporation and charge separation at the hot interface would serve to concentrate the precursor salt and in the same vicinity create local basic pH conditions owing to the counter hydroxide ion left behind after the loss of the hydronium ion to the vapours. The hydroxide ion would not only lead to the basic conditions required for a wide variety of nanoparticle formation [26] , [27] , [28] but it could also play a role as a reducing agent, [29] , [30] for instance, by discharging. Thus, a favourable environment for a cost-effective, efficient and green nanochemical reactor is created, as depicted in Fig. 1g . Faraday [31] was fascinated by the red colour of gold nanoparticles, which were synthesized by chemical reduction of a suitable gold precursor, such as AuCl 4 − ions with white phosphorus. Here we introduce the first experimental evidence of Leidenfrost chemical reactor that enables nanoparticle synthesis in a levitating drop without any additional reducing agent or sophisticated technique. For instance, a 2-ml drop of 10 mM aqueous Tetrachloroauric (III) acid solution (pH~2.3) was gently placed on a preheated hot plate, which was maintained at a temperature of 270 °C. A naked eye observation of a levitating drop of gold salts that converted to plasmonic red coloured gold nanoparticles is shown in Fig. 2a ( Supplementary Movie 4 ). At this stage, the drop was transferred to a commercial Lacey C/Cu grid, rinsed with hot water and subsequently dried in air for transmission electron microscopy (TEM) analysis, which revealed that the plasmonic colour arose from the formation of gold nanoparticles. 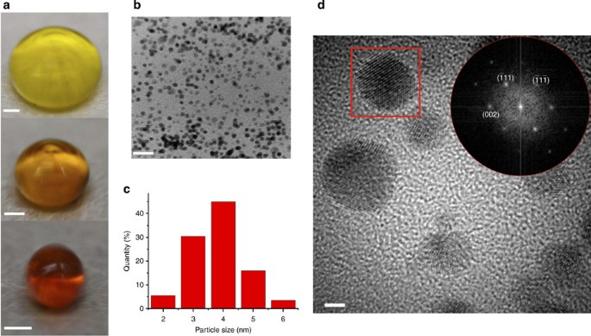Figure 2: Plasmonic gold nanoparticles using a levitating drop reactor. (a) Gold salts were converted to gold nanoparticles in a levitating drop without additional reducing agent and the drop slowly shrinks from a yellow plate-like disk into a red spherical droplet. Scale bar, 2 mm. (b) Bright-field TEM image recorded on the Au nanoparticles, scale bar, 20 nm and (c) particle size distribution. (d) High-resolution TEM micrograph with inserted fast Fourier transformation pattern calculated from the red marked region. The measured d-values of 0.237(5) nm, 0.235(5) nm and 0.207(5) nm are assigned to (11), (1) and (002) planes of Au, respectively. Zone axis [110], scale bar, 2 nm. Figure 2b depicts a bright-field TEM image recorded on the sample, which contains randomly oriented Au nanoparticles as proven by electron diffraction (not shown, the measured d -values are consistent with those from the literature [32] ). The histogram ( Fig. 2c ) depicts a narrow particle size distribution with an average diameter of ~4 nm. Occasionally, a few bigger nanoparticles were observed ( Supplementary Fig. S2 ). In addition, the high-resolution TEM images and fast Fourier transformation analysis reconfirms the presence of pure Au ( Fig. 2d ). The fast Fourier transformation pattern ( Fig. 2d , inset) of the square region containing a single Au nanoparticle ( cf . mark in Fig. 2d ) consists of the one expected for zone axis [110]. Figure 2: Plasmonic gold nanoparticles using a levitating drop reactor. ( a ) Gold salts were converted to gold nanoparticles in a levitating drop without additional reducing agent and the drop slowly shrinks from a yellow plate-like disk into a red spherical droplet. Scale bar, 2 mm. ( b ) Bright-field TEM image recorded on the Au nanoparticles, scale bar, 20 nm and ( c ) particle size distribution. ( d ) High-resolution TEM micrograph with inserted fast Fourier transformation pattern calculated from the red marked region. The measured d-values of 0.237(5) nm, 0.235(5) nm and 0.207(5) nm are assigned to (11), (1) and (002) planes of Au, respectively. Zone axis [110], scale bar, 2 nm. Full size image Scanning TEM–energy-dispersive X-ray (EDX) elemental maps (not shown) recorded on a similar region further support the presence of pure Au nanoparticles. When the experiment with the same reaction composition and conditions was carried out at lower temperature than the Leidenfrost ( Supplementary Fig. S3 ) or even in a conventional way (using oil bath at 100 °C), no nanoparticles were observed. Undoubtedly, our results prove that water under Leidenfrost conditions participates in and/or catalyses the chemical reaction, which is also supported analytically ( Supplementary Note 1 and Supplementary Fig. S4 ). Once the first clusters are formed, an autocatalytic pathway could set in where further ions are adsorbed and reduced on the surface of the metal clusters [33] . Nevertheless, our postulation need further investigations to explore the exact mechanism of the nanosynthesis. Nanosynthesis and three-dimensional coating in a Leidenfrost reactor The levitated chemical reactor suggested here can be used to fabricate metal oxide in the same manner. However, the technique is revolutionized when synthesis and coating occur simultaneously. One-pot synthesis and simultaneous coating of 3D objects is still a challenge for the bottom-up technique and is often a problematic task for nanofabrication in general [34] . Here, we introduce a levitated and rotating drop reactor for one-step synthesis and coating of a 3D object, e.g. TEM grid. As a demonstration, a 300 μl drop of 20 mM zinc acetate precursor solution (pH~6.3) was placed on a TEM grid, that was resting on a preheated (250°C) hotplate. 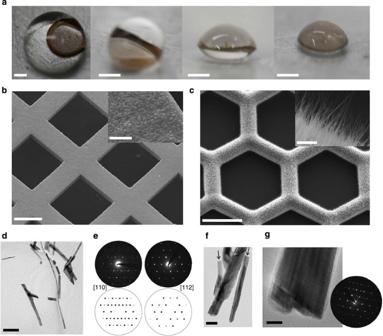Figure 3: Uniform coating of intricate three-dimensional substrates with ZnO nanoparticles and CuO nanorods. (a) TEM grid coated through Leidenfrost technique. TEM grid is completely covered by a levitating drop during the 3D coating process. Scale bar, 1 mm. (b) Scanning electron microscopy image of a TEM grid coated with (b) ZnO nanoparticles and (c) CuO nanorods. Inset shows the higher magnification of the coating. Scale bar of the image inbandc, 20 μm and 100 μm, respectively. Scale bar of the inset inbandc, 2 μm. (d) Bright-field image of several CuO nanorods. Scale bar, 200 nm. (e) Precession electron diffraction (PED) and selected area electron diffraction (SAED) patterns recorded on single nanorods with simulated patterns (based on the kinematic approximation). (f) Twinned nanorods with longitudinal twin boundaries,cf. arrows. Scale bar, 50 nm. (g) High-resolution micrograph of a twinned nanorod and SAED pattern. The rotation of the SAED pattern was adjusted according to the Fourier transform of the high-resolution micrograph, zone axis [011]. Scale bar, 10 nm. Figure 3a illustrates the drop levitation along with the TEM grid ( Supplementary Movie 5 ). Figure 3b depicts a scanning electron microscopy (SEM) micrograph of the TEM grid which has been coated three dimensionally with ZnO nanoparticles demonstrating a single one-pot synthesis and coating in a sterile and contamination-free environment using the Leidenfrost technique. EDX analysis at different regions of the sample ( Supplementary Fig. S5 ) showed that the chemical composition and the intensity ratio—which is very sensitive to any marginal change of the film thickness—are similar in different areas. Thicker coating with ZnO nanoparticles on other grid forms is also possible by increasing the concentration of the precursor (for example, 40 mM, pH ~6.2), ( Supplementary Fig. S6a ) or by multiple-steps coating ( Supplementary Note 2 and Supplementary Fig. S6b–f ). Figure 3: Uniform coating of intricate three-dimensional substrates with ZnO nanoparticles and CuO nanorods. ( a ) TEM grid coated through Leidenfrost technique. TEM grid is completely covered by a levitating drop during the 3D coating process. Scale bar, 1 mm. ( b ) Scanning electron microscopy image of a TEM grid coated with ( b ) ZnO nanoparticles and ( c ) CuO nanorods. Inset shows the higher magnification of the coating. Scale bar of the image in b and c , 20 μm and 100 μm, respectively. Scale bar of the inset in b and c , 2 μm. ( d ) Bright-field image of several CuO nanorods. Scale bar, 200 nm. ( e ) Precession electron diffraction (PED) and selected area electron diffraction (SAED) patterns recorded on single nanorods with simulated patterns (based on the kinematic approximation). ( f ) Twinned nanorods with longitudinal twin boundaries, cf . arrows. Scale bar, 50 nm. ( g ) High-resolution micrograph of a twinned nanorod and SAED pattern. The rotation of the SAED pattern was adjusted according to the Fourier transform of the high-resolution micrograph, zone axis [011]. Scale bar, 10 nm. Full size image Nanostructured coating of different materials in a rapid, cost-effective manner is routine by using this process. When copper acetate (~250 μl, 10 mM, pH~5.5) aqueous solution was used, CuO nanorods were fabricated ( Fig. 3c ). The number density, length and width of the rods can be manipulated by further heating (heated to 400 °C for 2 h) to produce CuO nanograss with micrometre length and a width in the range of tens of nanometres covering the surface ( Supplementary Fig. S6g ). EDX nanoprobe analyses confirmed the presence of Cu and O as the constituting chemical elements of the nanorods. Quantification of the EDX data recorded on several rods was consistent with an equimolar ratio of Cu and O within the experimental errors. The bright-field TEM image ( Fig. 3d ) shows several nanorods with high aspect ratios, including strongly bent species. The attached experimental and simulated diffraction patterns ( Fig. 3e ) recorded on single nanorods confirmed the assignment of the structure to the Tenorite-type [35] for the two zone axis (ZA) orientations [110] and [112], respectively. In the case of ZA [110], the precession electron diffraction mode was applied; thus, the dynamical scattering effects were considerably minimized. Many of the analysed crystals contained characteristic twins as recently described for CuO nanowires [36] , [37] . Twinning is indicated by longitudinal stripes in bright-field contrast microscopy ( Fig. 3f ), with boundaries running parallel to the (111) layer of the Tenorite-type structure. The twinning produces additional weak intensities between the high-intensity fundamental reflections ( Fig. 3g , inset shows the selected area electron diffraction pattern in the ZA [011]) by multiple scattering. Such phenomenon originates from a partial superposition of the twinned domains, and in this case the high-resolution contrasts exhibit clear modulation stripes as can be seen from Fig. 3g . The Leidenfrost dynamics (for example, large circulation current ( Supplementary Movie 5 )) and the stability of the loaded drop are crucial for a homogenous coating of the object. On the other hand, there are a number of experimental parameters and challenges, which influence the quality of the final structure such as surface roughness, wettability of the hot plate and the substrate to be coated, the geometric parameters of the substrate to be coated (for example, pinning by heterogeneity and defects). In addition, depending on the stability of the droplet, its rotation, deformation, vibration and oscillation, the final product will differ significantly and, consequently, the coating might face lack of uniformity. Moreover, probable sliding of the drop off the plate, the unbalanced substrate and other instability forms (that is, by bubble generation) could also ruin the feature of final structure ( Supplementary Fig. S7 ). Plasmonic nanoporous metal in a Leidenfrost pool Novel fabrication method of nanoparticles, their assembly and integration into practical devices are the main issues in the nanochemistry field. Nanoporous metal as a class of materials with a complex structure and wide variety of potential applications (see review by Bryce et al . [38] ), along with being outstanding candidates of plasmonic meta-materials with optical response determined by material constituents and porosity [39] , are difficult to be fabricated with traditional nanochemistry techniques [38] . Although top-down fabrication approaches, such as chemical etching and templating, are recognized as the methods of choice, they have their own disadvantages with respect to cost, yield, materials lost (that is, etching/removing the majority of the materials), requirement of hazardous chemicals, high temperatures and post activation. Wet chemical techniques, which are considered as a simple and low-cost alternative, have also serious drawbacks because of using hazardous chemicals/wastes, several processing steps and time consumption. Although the bottom-up wet chemical design of non-metallic porous structure has made enormous progress, it is still not well suited for metals [38] . In other words, finding a way for high yield of the metallic nanoparticles and their assemblies and agglomeration to form a 3D nanoporous structures is a difficult task, which cannot be performed with the traditional fabrication techniques. The Leidenfrost reactor is a unique phenomenon whose potential for technological application has not yet been explored. Here the Leidenfrost chemistry and Leidenfrost dynamics are combined and are potentially exploited as a new generator of 3D nanoporous metal. Achieving the mentioned task requires a production of concentrated aqueous nanoparticles inside the levitated droplet, which cannot simply be achieved by increasing the salt concentration for a good reason. Using only water for production of metallic nanoparticles, the Leidenfrost reactor is facilitated by the hydroxide ions, which promote both basic conditions and electron transfer reactions through discharging. Nevertheless, the yield is low, as the availability of the OH - ions is governed by the dissociation of water. According to our finding, the yield of the gold nanocrystals should increase, at least for higher concentrations of hydroxide ions. Herein, to meet the need of high concentrations, we further introduced a new type of reducing agent under the Leidenfrost condition, namely NaOH, as a source of hydroxide ions and enhancer of the basic condition. Indeed, by simply adding 50 μl of NaOH (0.5 M) to a 20 mM aqueous Tetrachloroauric (III) acid solution (pH~6.5) and gently placing a 5-ml drop of the resulting solution on a preheated hot plate (with a constant temperature of 270 °C), a brownish red droplet is formed, containing a dense structure. The structure was collected on a glass plate where a macroscopic spongy system can be seen even by the naked eye ( Fig. 4a ). 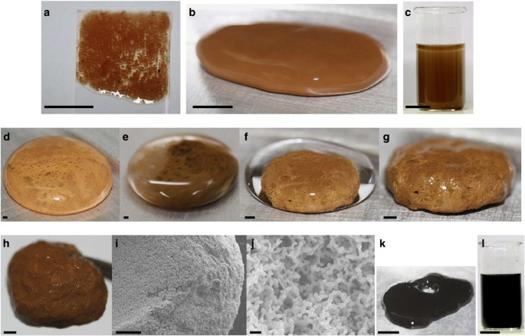Figure 4: Fabrication steps for nanoporous gold. (a) Photograph of spongy structure collected on a glass substrate using only NaOH. (b)Leidenfrost levitated pool of suspended nanoporous brown gold on hot plate. (c) The same solution as (b) collected inside a glass container. (a–c) Scale bar, 1 cm. Synthesis steps of solid nanoporous gold sphere from initialization (d) to final product as a sponge (e-h). Scale bar, 1 mm. (i) Scanning electron microscopy image of the spongy brown gold. Scale bar, 100 μm. (j) Higher magnification image of the same sample as ini. Scale bar, 300 nm. (k) Leidenfrost levitated pool of suspended nanoporous black gold on hot plate. (l) The same solution as (k) collected inside a glass container. (k,l) Scale bar, 1 cm. Figure 4: Fabrication steps for nanoporous gold. ( a ) Photograph of spongy structure collected on a glass substrate using only NaOH. ( b) Leidenfrost levitated pool of suspended nanoporous brown gold on hot plate. ( c ) The same solution as ( b ) collected inside a glass container. ( a – c ) Scale bar, 1 cm. Synthesis steps of solid nanoporous gold sphere from initialization ( d ) to final product as a sponge ( e - h ). Scale bar, 1 mm. ( i ) Scanning electron microscopy image of the spongy brown gold. Scale bar, 100 μm. ( j ) Higher magnification image of the same sample as in i . Scale bar, 300 nm. ( k ) Leidenfrost levitated pool of suspended nanoporous black gold on hot plate. ( l ) The same solution as ( k ) collected inside a glass container. ( k , l ) Scale bar, 1 cm. Full size image In our opinion, and from technological point of view, the field is revolutionized if 3D nanoporous structures could be fabricated in a suspension form, which would enable a simple casting-based device. To evaluate the potential of this idea, we sought out a way, to design and produce nanoporous metal in a suspension form. For that purpose, sodium citrate was used as a capping agent and simultaneously as a co-reducing agent beside the sodium hydroxide to further enhance the yield. On the basis of the mentioned approach, we demonstrate the first wet chemical synthesis of a suspended nanoporous gold using levitated Leidenfrost pool (1 ml HAuCl 4 , 20 mM+700 μl sod. citrate 1%+50 μl NaOH 0.5 M, pH~7.3) in a simple, cost-effective and green way ( Fig. 4b ). At this stage, a portion of the brown suspension was collected to glass bottles and stored for further use ( Fig. 4c ). Various analytical investigations (ultraviolet–visible spectroscopy for the liquid, as well as SEM and X-ray diffraction (XRD) on dried and rinsed samples) confirmed the formation of suspended plasmonic nanoporous gold (Supplementary Fig. S8). On the other hand, an orange suspension of a macroscopic 3D network of fused gold particles with different sizes and shapes are formed if only pure sodium citrate is used ( Supplementary Fig. S9 ). Gold suspension behaves analogous to polymer chains dispersed in a good solvent and it merely collapses to form a hard sphere upon solvent evaporation. A global evaporation of the levitated suspended gold pool acts very similar; however, it is expected that the gold chains are further fused and welded together to form a 3D nanoporous hard sphere. With that in mind, we further demonstrate an ‘all- in-situ ’ fabrication of 3D nanoporous hard sphere in the Leidenfrost drop. A naked eye observation of a levitating drop of the brown gold that converted into 3D nanoporous powder is shown in Fig. 4d–h . It is worth mentioning that the nanoparticle synthesis, clustering, assembly and fusion to form an extended 3D network occurred in the levitated drop. Washing, rinsing the sample and removing of residual salt and/or byproduct, or even enlarging the size of the metal spongy can occur ‘all- in-situ ” in the levitated state ( Supplementary Movie 6 ). SEM analysis proved the 3D macroporous structure of the gold sphere ( Fig. 4i,j and Supplementary Fig. S10 ), whereas the XRD pattern indicated the polycrystallinity of the sample (not shown). Our results demonstrate a new generation of metallic porous materials in a different form fabricated from a levitated drop and manifest the interplay between the Leidenfrost chemistry and Leidenfrost dynamics. To understand the origin of this phenomenon, we investigated the effect of Sod. hydroxide/Sod. citrate ratio as a possible variable on the structure. It is beyond the scope of this article to describe the details of all these experiments. But we can conclude that the shape, size, filling factor (porosity) and the plasmonic colour is highly affected by the added amount of NaOH and its concentration, whereas the stability of the suspensions is highly altered by the citrate content. Furthermore, our investigations implies the important role of this ratio on the heat transfer in the levitated drop, including the convective heat transfer performance of the nanofluids [40] , the evaporation in the levitated droplet, and the temperature and viscosity field around the particle, which affect its mobility, clustering and networking. Last but not the least, the ratio was found to be a determining factor controlling the place of spongy structure formation. In other words, depending on the ratio of hydroxide and citrate of sodium, the sponge is either likely to be formed mainly inside the droplet or mainly at the liquid–air interface in analogue to levitated liquid marbles [41] , [42] . We believe that a new multidisciplinary approach needs to be introduced to describe the interdependency between the Leidenfrost chemistry and Leidenfrost dynamics. It would not only enhance our understanding of the heat transfer phenomenon in a levitated droplet but also is essential for a new generation of tunable plasmonic porous materials. To visualize the role of NaOH mentioned above and to further explore the potential of the mentioned method, we demonstrate the first black gold suspended in a levitated pool ( Fig. 4k ) and collected in a glass bottle ( Fig. 4l ). The black gold suspension, which we believe to cause a paradigm shift in the field of plasmonics, has been fabricated by increasing the amount of hydroxide ions, that is, NaOH to 150 μl, while keeping all the other parameters required for the fabrication of the brown gold suspension constant (1 ml HAuCl 4 , 20 mM+700 μl Sod. citrate 1%+150 μl NaOH 0.5 M, pH~8.5). A full analytical investigation of the resulting black product was performed (see Supplementary Figs S11 and S12 ). We believe that our black nanoporous suspension fabricated under Leidenfrost condition can turn any substrate to a super absorber by simple casting, and hence enable a new generation of functional plasmonic that can be easily integrated in several energy collecting application, including photovoltaics and thermo-photovoltaics. Although an up-to-date achieving black absorber are mainly based on top-down approaches, such as focused ion beam [43] , lithography [44] and co-sputtering [45] , which are comparably costly and their absorption band limited to the visible spectrum, here we demonstrate the first casting-based wideband superabsorber with almost 100% absorbance covering visible to the telecommunication wavelength. This new type of black coating can be applied onto any kind of substrates, including flexible ones ( Fig. 5a ) with a thickness of ~20 μm ( Fig. 5b ). As the transmission of such a film is zero, the absorption can be calculated by measuring the reflectance of the samples (absorption=1−reflection). Spectroscopy measurement showed that the reflectance of the black spongy gold is almost zero in whole, visible up to 2 μm wavelength and, hence, resulting in almost 100% absorbance in that frequency regime ( Fig. 5c ). We believe that the suppression of light reflection originated through combined effects of strong scattering of the light by the sample roughness, localized and de-localized excitation of plasmon within and on the surface of pores, as well as light trapping inside the gaps. In addition to being a superabsorber, the cast film exhibits a pretty high conductivity of 7.958 × 10 3 S m −1 and, hence, can function as a new type of window electrode in the photovoltaic device [46] . 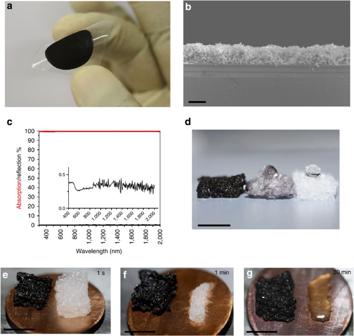Figure 5: Function-based black nanoporous gold. (a) A flexible polymeric substrate coated with the black spongy gold. (b) Cross sectional scanning electron microscopy image of black spongy gold showing the thickness of film ina. Scale bar, 20 μm. (c) Reflection and absorption spectra of black spongy gold in the visible and near-infrared frequency. Inset shows the magnified reflection spectra in the same frequency. (d, Left of panel) Plastic foam coated with black gold in Leidenfrost levitated drop showing superhydrophilic behaviour. (Middle of panel) Plastic foam immersed in black gold solution for 24 h showing hydrophobic behavior. (Right of panel) Neat plastic foam showing hydrophobic behaviour. Heating stages of coated (black) and neat foam (white) on a hot plate after (e) 1 s, (f) 1 min and (g) 30 min at 150 °C (d–g). Scale bar, 1 cm. Figure 5: Function-based black nanoporous gold. ( a ) A flexible polymeric substrate coated with the black spongy gold. ( b ) Cross sectional scanning electron microscopy image of black spongy gold showing the thickness of film in a . Scale bar, 20 μm. ( c ) Reflection and absorption spectra of black spongy gold in the visible and near-infrared frequency. Inset shows the magnified reflection spectra in the same frequency. ( d , Left of panel) Plastic foam coated with black gold in Leidenfrost levitated drop showing superhydrophilic behaviour. (Middle of panel) Plastic foam immersed in black gold solution for 24 h showing hydrophobic behavior. (Right of panel) Neat plastic foam showing hydrophobic behaviour. Heating stages of coated (black) and neat foam (white) on a hot plate after ( e ) 1 s, ( f ) 1 min and ( g ) 30 min at 150 °C ( d – g ). Scale bar, 1 cm. Full size image Hybrid foam in a levitated Leidenfrost drop The uniqueness and power of Leidenfrost drop as a nanogenerator, nanocoater and nanodesigner of functional porous materials is further revealed by the fabrication of a functional metal–polymer hybrid foam. By introducing a commercial packaging polymer foam in a levitated black pool, a black metal–polymer hybrid foam is generated ( Fig. 5d (left)). However, if the polymer foam is immersed onto a glass bottle containing the black suspension for 24 h at room temperature, or even immersed and then followed by evaporation of the solvent, the foam cannot be coated totally to realize a black hybrid foam ( Fig. 5d (middle)). Thus, a 3D coating of complex structure can be only performed under the Leidenfrost dynamics, which further shows the uniqueness of this phenomenon for nanocoating processes. However, covering an area larger than the porous template demonstrated in this study is a challenge. In other words, as the deformation and stability threshold of the levitated droplet is size-limited [14] , coating any object bigger than the size of a stable droplet is unattainable. It is worth mentioning that the fabricated hybrid foam is stable even after repeated washing and air-drying ( Supplementary Fig. S13 ). In contrast to its neat counterpart, the hybrid foam is superhydrophilic ( Fig. 5d ), thanks to the high energy porous metal coating. Indeed, the applications of this type of hybrid foam are too numerous to ascertain, one of the most potential uses is in areas where good heat dissipation, low thermal expansion and light weight are needed (for example, electronic packaging and aerospace). As a proof of concept and only to visualize this effect, placing the foam on the hot plate of 150 °C along with a bare foam showed that stability of the foam is significantly improved because of the metallic coating. Figure 5e–g shows the sequence of heating where one can see that the neat foam melted, while the hybrid one maintained its shape due to its metallic-like heat dissipation. Indeed, the black hybrid foam shows a wideband superabsorber behaviour similar to the casted black gold on the polymer foil (not shown). As the colour of porous plasmonic meta-materials is dictated by the size of the pores [47] , it is expected that the colour difference of the black (spongy/hybrid) and the brown gold originates from the dissimilarity of the average pore size. BET (Brunauer–Emmett–Teller) analysis of the spongy brown, black and hybrid foam ( Supplementary Fig. S14 and Supplementary Table S1 ) proved that the black porous spongy and the black hybrid possessed a nearly similar average pore size of ~2.6 and 2.4 nm, respectively, whereas the brown porous gold has an average pore diameter that exceeded 3 nm. All in all, we believe that our work has contributed to resolve the 257-year-old Leidenfrost phenomenon, while we prove the electrostatic, thermal gradient and overheated nature of the levitated droplet. The later already manifest our hypothesis of the overheated zones [2] and we believe that a new type of charge chemistry has been introduced and the effectiveness of the Leidenfrost drop as a water-based levitated green reactor for nanochemistry along with the extensive usefulness of implementation of its exclusive physiochemical character has been demonstrated. Nevertheless, the exact mechanism of the nanosynthesis, including the role of the fast evaporation and thermocapillary, is still unknown and has to be determined. Lab in a Leidenfrost drop allows the fabrication of nanomaterials and simultaneously implementing it for the designing of functional materials by a fast one step, low cost and in an environment-friendly manner, all in a levitated drop. Especially noteworthy is the designing of plasmonic nanoporous gold in suspension form that allow to demonstrate the first bottom-up-based wideband black absorber. The 3D coating of a complex structure performed under the Leidenfrost dynamics further shows the uniqueness of this phenomenon for nanocoating processes. However, although small objects can be coated, covering big object is limited to the biggest droplet that can levitate stably under the Leidenfrost condition. In this context, the uniformity and the quality of the coating is influenced by several parameters, such as surface roughness, wettability of the hot plate and the substrate to be coated, and the geometrical factors, which hinder the movement of the droplet or affect its shape, stability and vibration. Nevertheless, and as was mentioned in previous work [2] , the Leidenfrost drop may be able to maintain a metastable state, although this requires further investigation to be proved. In short, the Leidenfrost reactor has just started and is full of interesting problems that require multidisciplinary investigations to fully understand the phenomenon and to explore the interdependency between the Leidenfrost chemistry, Leidenfrost dynamics and heat transfer phenomenon in a levitated droplet. TEM and SEM characterizations TEM measurements were carried out using an FEI/Philips Tecnai F30 G2 TEM (FEG cathode, 300 kV, C s =1.2 mm) equipped with EDX detector and Gatan imaging filter, and with a Philips CM 30ST microscope (LaB 6 cathode, 300 kV, C s =1.15 mm). A Spinning Star device (Nanomegas) attached to the CM 30 microscope enabled precession electron diffraction. Thin films were mechanically released to Cu lacey carbon TEM grids by scratching and mixing with Butanol for enhancing adhesion. For the case of CuO nanorods, a Mo TEM grid was used. SEM measurements were carried out using a Phillips XL 30 and a Field Emission SEM ZEISS ULTRA plus equipped with Oxford Instruments INCA-X-act EDS. Ultraviolet–visible/NIR spectroscopic analysis The reflection and absorbance spectra of black and brown gold nanoparticles ( Fig. 5c and Supplementary Fig. S8b and S11c ) were investigated by Lambda900 UV/vis/NIR spectrometer (Perkin Elmer). Aluminum mirror were used as a standard for the reflectance measurement, while the standard cuvette was utilized for the solution measurements. Electrical conductivity measurements The conductivity of black Au film, cast on the plastic substrate, was determined by a Keithley 6517B electrometer and ‘National Instruments LabView’ software. A constant voltage of 1 V was applied between two Au-wire electrodes located on the film sample (width of electrodes, w =0.3 mm and the distance between the electrodes, d =2 cm). BET, XRD and infrared imaging investigation Porosity and surface-area characterization for brown, black gold and hybrid foam samples are done by a BELSORPmax machine from Rubotherm. All XRD measurements were carried out by a Seifert XRD 3000 PTS. InfraTec PIR uc 180 with a rate of 24 Hz and a spatial resolution of 40 lm/IR pixel was used for thermographic analysis of the levitated drop. How to cite this article: Abdelaziz, R. et al . Green chemistry and nanofabrication in a levitated Leidenfrost drop. Nat. Commun. 4:2400 doi: 10.1038/ncomms3400(2013).